Photon-enhanced thermionic emission from heterostructures with low interface recombination Photon-enhanced thermionic emission is a method of solar-energy conversion that promises to combine photon and thermal processes into a single mechanism, overcoming fundamental limits on the efficiency of photovoltaic cells. Photon-enhanced thermionic emission relies on vacuum emission of photoexcited electrons that are in thermal equilibrium with a semiconductor lattice, avoiding challenging non-equilibrium requirements and exotic material properties. However, although previous work demonstrated the photon-enhanced thermionic emission effect, efficiency has until now remained very low. Here we describe electron-emission measurements on a GaAs/AlGaAs heterostructure that introduces an internal interface, decoupling the basic physics of photon-enhanced thermionic emission from the vacuum emission process. Quantum efficiencies are dramatically higher than in previous experiments because of low interface recombination and are projected to increase another order of magnitude with more stable, low work-function coatings. The results highlight the effectiveness of the photon-enhanced thermionic emission process and demonstrate that efficient photon-enhanced thermionic emission is achievable, a key step towards realistic photon-enhanced thermionic emission based energy conversion. Advancing the efficiency of solar-energy harvesting beyond the Shockley–Queisser limit has been the holy grail of the solar-energy field since the publication of their landmark paper in 1961 (ref. 1 ). A number of new concepts and novel physical mechanisms have been proposed to overcome this limit on single-junction solar cells, including multi-junction cells [2] , [3] , multiple exciton generation [4] , [5] and hot-carrier harvesting [6] , [7] , all of which aimed at avoiding the thermalization and absorption losses inherent in conventional photovoltaic cells. Investigations into hot-carrier conversion have typically focused on highly non-equilibrium carrier collection, which aims to extract photoexcited carriers at elevated kinetic energy much more quickly than they can lose energy via thermalization with the lattice [7] , [8] . The efficiency of such a hot-carrier cell can theoretically approach the thermodynamic limit for solar-energy conversion of ~85% (ref. 7 ). However, thermalization, driven by electron-phonon interactions, is usually a very fast process on the order of picoseconds, and slowing it to a rate that allows efficient charge collection at elevated electron energies remains a challenge in material physics [9] , [10] . Recently, a new concept has been proposed for high-temperature electron harvesting. Photon-enhanced thermionic emission (PETE) is based on vacuum emission of photoexcited electrons that are in thermal equilibrium with a hot semiconductor’s lattice [11] . As electrons and the lattice are at the same temperature, the rate of electron extraction in the PETE process does not need to compete with thermalization (as it does in hot-electron harvesting), but instead must simply exceed the rate of recombination. Recombination between bands can be orders of magnitude slower than thermalization within bands, making PETE a promising route to efficient high-temperature electron conversion. Although theoretically expected to have high efficiency, proof-of-concept measurements of the PETE process on thin-film GaN displayed very low quantum efficiencies, on the order of 10 −4 –10 −3 electrons per incident photon [11] . These efficiencies are too low for most practical applications and lower than conventional photocathodes [12] , [13] , [14] . Emission due to PETE in these experiments was obscured by competing photoemission mechanisms and by other complications associated with the emission process, including non-equilibrium transport through the surface band-bending region. As a result, only qualitative descriptions of PETE were made, and the underlying physical reasons for the measurements’ low emission efficiency have remained poorly understood. Here we describe a heterostructure architecture designed to decouple the basic physics of PETE from the vacuum emission process. By separating PETE from the photoemission mechanisms that complicated earlier proof-of-concept measurements, we are able to directly compare theoretical expectations to experimental results. Our measurements show a dramatic improvement in experimental PETE quantum efficiency over previous experiments due to reduced recombination at the internal heterointerface, representing a major step for the prospects of solar-energy conversion based on PETE. Electron emission from a heterostructure cathode The heterostructure cathode is based on two layers, an absorber material and a nanoscale emitter layer with a larger band gap, as shown in Fig. 1 . Photons excite electrons into the absorber’s conduction band, which then rapidly thermalize and diffuse throughout the absorber. When the electrons encounter the junction with the emitter, a fraction of them have sufficient thermal energy and enter the emitter’s conduction band, from which they can then continue into vacuum. In a device, these electrons are then collected by a second electrode at lower temperature called the anode, generating current. The ideal output voltage in a PETE device is the difference in work functions between the anode and cathode. 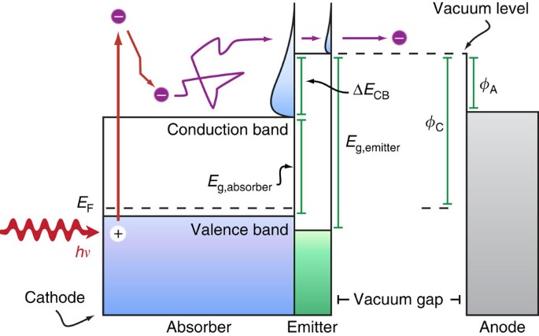Figure 1: Simplified band diagram showing a PETE device with a heterostructure cathode. The cathode is separated by a vacuum gap from an anode at lower temperature and lower work functionφA. PETE in the cathode occurs in three steps: photoexcitation, transport and emission. The heterostructure splits the emission step in two: internal PETE and external photoemission. The band gaps are denoted byEg,absorberandEg,emitter, the difference in energy between the conduction band minima in the absorber and nanoscale emitter is ΔECB, and schematic thermal distributions are shown at both the absorber/emitter interface and at the emitter/vacuum interface. The cathode’s work functionφCis the difference between the cathode Fermi levelEFand the vacuum level at the emissive surface. This article focuses on the cathode side of the device, examining a heterostructure based on GaAs coated with Cs-O to lower its work function. Figure 1: Simplified band diagram showing a PETE device with a heterostructure cathode. The cathode is separated by a vacuum gap from an anode at lower temperature and lower work function φ A . PETE in the cathode occurs in three steps: photoexcitation, transport and emission. The heterostructure splits the emission step in two: internal PETE and external photoemission. The band gaps are denoted by E g,absorber and E g,emitter , the difference in energy between the conduction band minima in the absorber and nanoscale emitter is Δ E CB , and schematic thermal distributions are shown at both the absorber/emitter interface and at the emitter/vacuum interface. The cathode’s work function φ C is the difference between the cathode Fermi level E F and the vacuum level at the emissive surface. This article focuses on the cathode side of the device, examining a heterostructure based on GaAs coated with Cs-O to lower its work function. Full size image The clean division between internal PETE and external emission in a heterostructure cathode offers several advantages. At the internal absorber/emitter interface, the barrier to PETE can be conveniently tuned by the offset in the emitter and absorber conduction band minima Δ E CB . In contrast, the energy barrier at the emitter/vacuum interface can be minimal, allowing the emitter/vacuum interface to be independently studied and optimized for efficient emission into vacuum. Importantly, these interfaces can be effectively decoupled with an emitter thickness less than ~100 nm, which is on the order of the electron mean-free path in common high-quality semiconductors [15] . As a result, electrons can travel through the nanoscale emitter with minimal scattering (and recombination) before encountering the band-bending region at the emitter/vacuum interface. Furthermore, as will be seen in this article, the reduced recombination at the internal interface can dramatically increase the effectiveness of the PETE process, making PETE far more appealing for practical applications. The heterostructure simplifies analysis by separating PETE from competing photoemission mechanisms in photon energy. The three relevant emission mechanisms are illustrated in Fig. 2a . In the PETE process (i), electrons excited in the absorber conduction band ( hv > E g,absorber ) first thermalize to the lattice temperature. However, as shown in Fig. 2a , if photons incident on the absorber have sufficient energy ( hv > E g,absorber +Δ E CB ), a fraction of photoexcited electrons can escape into the emitter before complete thermalization with the lattice, giving rise to internal photoemission (ii). Finally, photons with energies greater than the emitter’s band gap ( hv > E g,emitter ) can generate band-to-band transitions within the emitter, resulting in direct photoemission (iii). The two photoemission processes, internal photoemission before thermalization and direct photoemission from the emitter, require greater photon energies than needed for PETE. As a result, for photons with energies close to the absorber’s band gap hv ≈ E g,absorber , emission is due exclusively to PETE. 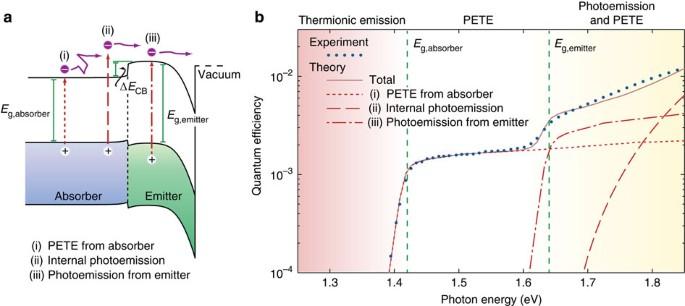Figure 2: Regimes of electron emission into vacuum from the heterostructure cathode after activating with Cs and O to lower the work function. (a) Illustration of the competing emission mechanisms: (i) PETE from the absorber, (ii) internal photoemission from the absorber before complete thermalization and (iii) direct photoemission into vacuum from the nanoscale emitter. Photoemission before thermalization is shown from the absorber but some are possible from other sources, for example, from the band-bending region of the emitter. The band diagram is calculated with PC1D for the GaAs/Al0.15Ga0.85As heterostructure studied here, and the band gaps and absorber thickness are decreased for illustration. (b) Experimental (blue curve) and calculated (red curves) quantum efficiency as a function of photon energy. The band gaps of the absorberEg,absorberand emitterEg,emitterare shown as vertical dashed green lines. Figure 2: Regimes of electron emission into vacuum from the heterostructure cathode after activating with Cs and O to lower the work function. ( a ) Illustration of the competing emission mechanisms: (i) PETE from the absorber, (ii) internal photoemission from the absorber before complete thermalization and (iii) direct photoemission into vacuum from the nanoscale emitter. Photoemission before thermalization is shown from the absorber but some are possible from other sources, for example, from the band-bending region of the emitter. The band diagram is calculated with PC1D for the GaAs/Al 0.15 Ga 0.85 As heterostructure studied here, and the band gaps and absorber thickness are decreased for illustration. ( b ) Experimental (blue curve) and calculated (red curves) quantum efficiency as a function of photon energy. The band gaps of the absorber E g,absorber and emitter E g,emitter are shown as vertical dashed green lines. Full size image Modelling PETE In this intermediate photon-energy regime, PETE dominates and can be directly compared with theoretical expectations. On the basis of a model we have developed for the PETE process [16] , the rate of PETE can be described using an emission velocity S PETE , analogous to a recombination velocity at the absorber/emitter interface: Here v x is the average thermal velocity of electrons perpendicular to the material’s surface, k B is the Boltzmann constant, T is the sample temperature and R e is the average probability of electron reflection either at the absorber/emitter interface or due to scattering within the emitter. The thermal velocity v x sets the rate at which electrons encounter the absorber/emitter interface, whereas (1− R e ) × exp(−Δ E CB / k B T ) represents the probability that the electrons continue into the emitter. The quantum efficiency is dependent on a simple competition between this PETE velocity (equation 1) and recombination [16] : In this equation, S 1 is the recombination velocity at the absorber/emitter interface, and recombination in the bulk and at the back surface is encapsulated by , where D is the diffusion coefficient, L is the diffusion length, d is the thickness of the absorber and is a dimensionless parameter that quantifies the change in recombination due to the inclusion of a back surface with the recombination velocity S 2 . The probability that an electron travels through the emitter’s band-bending region and into vacuum without recombining is incorporated into a factor b , similar to typical treatments of negative electron-affinity photoemission [12] . The final term A = A ( α , d , L , ζ 2 ) represents the fraction of photons absorbed and the effects of the photoexcited electrons’ initial spatial distribution for an absorption coefficient, α . Further detail can be found in the Supplementary Methods . These factors, b and A , translate the internal competition between PETE and recombination into an external efficiency, allowing this relation to be used to model experimental results. Room-temperature measurements Figure 2b displays a characteristic quantum efficiency curve at ~30 °C from a heterostructure grown by molecular beam epitaxy. Here the absorber layer is 1 μm GaAs, the emitter is 70 nm Al 0.15 Ga 0.85 As, and a backing layer of 100 nm Al 0.4 Ga 0.6 As forms a boundary for electrons diffusing within the absorber. All layers are 10 18 cm −3 Be-doped, minimizing the energy difference between the absorber and emitter valence bands ( Fig. 2a ) and resulting in a nearly temperature-independent energy barrier Δ E CB ≈0.22 eV (refs 17 , 18 , 19 ). This barrier is approximately the difference in absorber and emitter band gaps, increasing the energy onset of internal photoemission from the absorber ( hv > E g,absorber +Δ E CB ) to coincide with the start of photoemission from the emitter ( hv > E g,emitter ). After a 1-min treatment in 9% HCl, the sample is loaded into vacuum and heated to prepare the surface. To lower the work function, the sample is then activated with Cs and O 2 , a coating used extensively in photocathode applications [12] , [20] . The emission in Fig. 2b falls into distinct regimes based on photon energy, separated by the band gaps of the absorber and emitter (vertical dashed green lines). In the lowest energy region ( hv 1.42eV), photons have insufficient energy to excite band-to-band transitions in either the absorber or the emitter, and emission, which might have been due to defects or thermal means, is minimal. In the middle region (1.42eV hv 1.64eV), photons can excite electrons within the absorber layer but not the emitter, and emission is dominated by PETE. Finally, in the third region photons have energies in excess of the emitter band gap ( hv 1.64eV), and the current is due to both PETE and photoemission. The theoretical PETE yield calculated from equation 2 is shown in Fig. 2b as a dotted red line, using literature values for absorption [21] , [22] , transport [17] and radiative recombination [23] in p-type GaAs. The contributions of the two photoemission mechanisms using typical theoretical models are shown as dash-dotted and dashed lines [12] , [24] . The sum of all three emission mechanisms (solid) displays good agreement with the experimental data (blue). The minor differences at higher photon energies are primarily due to the simplicity of the emitter photoemission model. Additional modelling details can be found in the Supplementary Methods . The primary interest of this work is the intermediate photon-energy regime, where emission is dominated by PETE. In this regime, the shape of the theoretical quantum efficiency curve matches the experimental data very well, highlighting the effectiveness of equation 2 in modelling the PETE process in this heterostructure. However, it should be noted that the magnitude of this theoretical quantum efficiency depends on some device-dependent parameters in the model (for example, b , S 1 , S 2 ), which have competing or correlated effects on overall emission. Although these device-dependent parameters cannot be uniquely determined from the quantum-efficiency curves, it is nonetheless possible to put approximate bounds on their magnitudes by ensuring that the overall theoretical emission agrees well with experimental results. Using these constraints, the interface recombination velocities S 1 and S 2 in this sample can be estimated to be at most ~10 4 cm s −1 . This suggests that bulk recombination dominates in this heterostructure [16] . Indeed, the interface recombination velocities S 1 and S 2 could be much lower than 10 4 cm s −1 and fit experimental data well. Recombination rates on this order are not uncommon at high-quality heterointerfaces, which can achieve recombination velocities lower than 10–100 cm s −1 (refs 25 , 26 , 27 ), but are considerably better than those seen at the surfaces of p-type semiconductors, which can exhibit velocities on the order of ~10 6 –10 7 cm s −1 (refs 28 , 29 , 30 ), close to the electron thermal velocity. In calculations shown in Fig. 2 and elsewhere, the interface recombination velocities are at this approximate maximum of 10 4 cm s −1 to conservatively estimate the efficiency of the internal PETE process. These interface recombination velocities imply a probability of emission through the emitter’s band-bending region of b ≈0.25 to match experimental data. This low fraction is common in photocathode applications [20] , as recombination at Cs-O-coated semiconductor surfaces is typically not better than at bare surfaces. Although emission efficiency could still be increased up to approximately four times by reducing emissive-surface recombination, the results here highlight a critical advantage of the heterostructure architecture. Owing to the internal energy barrier at the absorber/emitter interface, electrons encounter the emissive surface far fewer times than they would in a cathode without an emitter layer. As a result, electrons have far fewer opportunities to recombine at the emissive surface. This can dramatically increase emission efficiency, as the requirements on emissive-surface recombination are considerably lower. For comparison, if the recombination velocity at the internal absorber/emitter interface were at the high level of ~10 6 –10 7 cm s −1 rather than 10 4 cm s −1 , PETE in Fig. 2b would be expected to be one to two orders of magnitude less efficient. Temperature-dependent measurements In addition to increasing the room-temperature efficiency, reduced interface recombination is also expected to increase the efficiency’s temperature dependence, as a smaller increase in emission probability is needed to overcome the competing recombination mechanisms in equation 2. The effect of temperature on the experimental quantum efficiency from this heterostructure is shown in Fig. 3a . As the sample is heated from ~30 °C to ~120 °C (blue to dark red), the measured quantum efficiency in the PETE region displays a dramatic increase of an order of magnitude, from ~0.16% to 1.4% at 1.5 eV (850 nm). These results represent an exceptional increase in PETE efficiency over previous measurements [11] . Impressively, as temperature increases the distinction between the PETE regime and the photoemission regime essentially disappears, as electrons overcome the energy barrier more efficiently, and PETE begins to dominate the overall emission current. 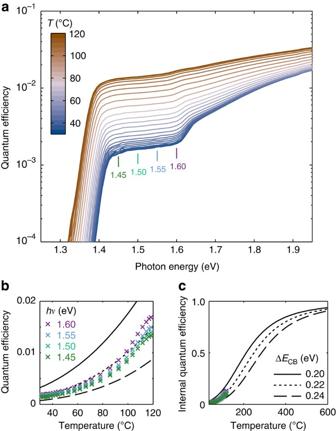Figure 3: Effect of temperature on experimental PETE quantum efficiency. (a) As temperature increases (blue to dark red), experimental PETE quantum efficiency increases by an order of magnitude. (b) Experimental quantum efficiency as a function of temperature for photon energies between 1.45 and 1.60 eV, as marked ina. Theoretical temperature dependences for three barrier heights 0.20, 0.22 and 0.24 eV are shown in black as solid, dotted and dashed lines. (c) Internal PETE quantum efficiency at the absorber/emitter interface extrapolated to higher temperature. Figure 3: Effect of temperature on experimental PETE quantum efficiency. ( a ) As temperature increases (blue to dark red), experimental PETE quantum efficiency increases by an order of magnitude. ( b ) Experimental quantum efficiency as a function of temperature for photon energies between 1.45 and 1.60 eV, as marked in a . Theoretical temperature dependences for three barrier heights 0.20, 0.22 and 0.24 eV are shown in black as solid, dotted and dashed lines. ( c ) Internal PETE quantum efficiency at the absorber/emitter interface extrapolated to higher temperature. Full size image The measured quantum efficiency of 1.4% at ~120 °C corresponds to an internal quantum efficiency of the PETE process itself at the absorber/emitter interface of at least ~(7–10)% ( Supplementary Methods ). However, even at this temperature the barrier Δ E CB ≈0.22 eV is around six times the thermal energy k B T , giving a probability of escape into the emitter of only exp(−Δ E CB / k B T )≈0.2%. Thus, on average, an electron collides with the interface with the emitter 500 times before it has sufficient thermal energy for emission. In contrast, at least ~(7–10)% of electrons excited in the absorber escape into the emitter using PETE, demonstrating the quality of the absorber/emitter interface. The temperature dependence of the quantum efficiency is shown in Fig. 3b for photon energies between 1.45 and 1.60 eV. As expected for PETE, where photoexcited electrons are assumed to thermalize before emission, the dependence is not strongly affected by the energy of the incident illumination. This is in contrast to photoemission before complete thermalization, where the quantum efficiency is closely tied to the initial kinetic energy of photoexcited electrons and roughly has a power-law dependence on incident photon energy [24] . Also shown in Fig. 3b are calculated quantum efficiencies at a photon energy of 1.5 eV for energy barriers of 0.20 eV (solid line), 0.22 eV (dotted line) and 0.24 eV (dashed line). The theoretical curves include a reduction of the radiative recombination coefficient [31] and a change in absorption coefficient due to the shift of band gap with temperature [19] . The experimental temperature dependence closely follows the theoretical prediction for the expected energy barrier of Δ E CB ≈0.22 eV. The temperature range in these experiments is limited by the stability of the low work-function Cs-O coating. Cs-based coatings are not as stable on GaAs-based materials [32] as on the GaN samples used in previous experiments, and the coating here degrades over time and at elevated temperatures. To minimize this deterioration, the sample temperature in Fig. 3 is kept below ~120 °C ( Supplementary Fig. S1 ), around 100 °C lower than measurements on GaN [11] . The data in Fig. 3 are furthermore taken as temperature rises (and before the coating eventually evolves into a positive electron-affinity barrier) to eliminate any apparent increase of temperature dependence related to coating degradation. Projecting the internal quantum efficiency to higher temperatures in Fig. 3c , if Cs-O were replaced with a coating stable to 300–500 °C, PETE efficiencies an order of magnitude higher than those reported here (and over 70% internally) could be readily achieved from the same sample. Temperatures in this range would also be much more relevant for solar conversion applications in tandem with solar thermal devices, where the ‘cool’ anode could be expected to be 300 °C or higher [11] . Furthermore, although the heterostructure architecture reduces requirements on recombination at emissive surface, emissive-surface recombination nonetheless limits the external quantum efficiency here (and in similar GaAs-based photocathodes [20] ) to, at most, ~25–50%. Therefore, emission from these heterostructures is limited by the current coating, which can be optimized separately in future work, and not by the effectiveness of the internal PETE physics. These results establish that the PETE process is not fundamentally restricted to low efficiencies but could form the basis of practical devices. Measurements reported here suggest that interface recombination is both dramatically reduced compared with previous work on bare semiconductors and significantly lower than the rate of bulk recombination in the absorber. This is a critical comparison for optimizing high-efficiency devices, as surface recombination must be lower than bulk recombination not to be the limiting factor in emission from a PETE cathode. Bulk recombination can be reduced in future work by using thinner absorbers and with better light trapping [16] . These improvements to photon management, along with the ultra-low interface recombination velocities possible in heterostructures [25] , [26] , [27] , illuminate a path to PETE devices with very high emission efficiencies. Remarkably, the emission efficiencies at the low measurement temperatures here are already approaching the quantum efficiencies of GaAs activated to a state of negative electron affinity, which can display quantum efficiencies >10% for photons with energies near the band edge [12] , [13] , [14] . As a result, PETE cathodes could potentially replace conventional photocathodes, particularly in situations requiring photosensitivity at energies close to or lower than easily achievable work functions. Electrons emitted from these heterostructures overcome an energy barrier greater than 0.2 eV. This thermal energy is unusable in conventional, Shockley–Queisser-limited photovoltaic cells, but in a PETE converter it would directly contribute to operating voltage. Large operating voltages are key to achieving the impressive conversion efficiencies theoretically predicted for PETE devices [11] , and would be enabled with even larger energy barriers than used in this heterostructure. The substantial improvement in quantum efficiency seen in this heterostructure represents a major step for the prospect of realistic devices based on PETE. Heterostructure growth and preparation The heterostructure was grown on a p-doped GaAs substrate using solid-source molecular beam epitaxy. The heterostructure consists of a 100-nm p-doped Al 0.4 Ga 0.6 As layer, a 1-μm p-doped GaAs layer and a 70-nm p-doped Al 0.15 Ga 0.85 As layer. All layers were uniformly doped with Be to a doping density of 10 18 cm −3 . A sample was cleaved from the wafer and sonicated in acetone, methanol and isopropanol for 10 min each. The sample was then loaded into a N 2 glovebox and treated in 9% HCl for 1 min followed by two 1-min rinses in deionized water before being placed onto a sample holder and being loaded into vacuum. After transfer into the main experimental chamber (base pressure <2 × 10 −10 Torr), the sample was heated to ~450 °C for 30 min. Activation and measurement After cooling, the sample was activated near room temperature to a peak in photocurrent using Cs (Alvatec Cs-Bi source), and then further activated with both Cs and O 2 until the photocurrent peaked again. The sample was then repeatedly cycled in temperature from ~120 to ~30 °C and back to ~120 °C, with each cycle lasting approximately 6 h, as shown in Supplementary Fig. S1 . Temperature-dependent data reported here were measured during the increase from ~30 to ~120 °C in the first cycle. The sample was illuminated with a monochromatized 150 W Xe lamp. A biased electrode in the vacuum system accelerated electrons away from the sample. Temperatures reported here are directly measured from the shift in band gap from the quantum efficiency curves using the well-known Varshni relation [19] , as a reference thermocouple did not match the sample temperature as well as it did in previous measurements [11] owing to modifications to the heater assembly. These temperatures are expected to be accurate to ±5 °C over the experimental range. A dditional information How to cite this article: Schwede, J. W. et al. Photon-enhanced thermionic emission from heterostructures with low interface recombination. Nat. Commun. 4:1576 doi: 10.1038/ncomms2577 (2013).